Alternative lengthening of telomeres is not synonymous with mutations in ATRX/DAXX 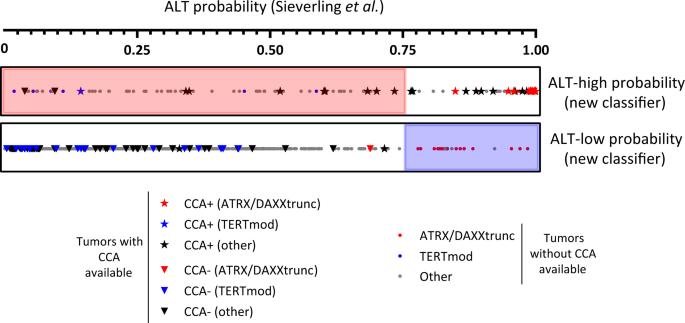Fig. 1: Comparison of the ALT-probability score of Sieverling et al.2, with the new classifier proposed in this article. The 2497 patients described in Sieverling et al. are divided here into two groups: ALT-high probability (upper bar) and ALT-low probability (lower bar) according to the new classifier. Within the two bars, each patient is represented by a symbol placed on a scale from 0 to 1 according to its Sieverling ALT-probability score. Star and inverted triangle symbols represent patients whose tumors were C-circle assay (CCA) positive or negative, respectively3, and the dots represent patients for whom CCA data are unavailable. Red and blue symbols correspond to patients with ATRX/DAXXtrunc and TERTmod alterations, respectively2. The pink and blue shading highlights the tumors for which the two scores were discordant: the pink shading in the upper box indicates tumors with ALT-high probability (new classifier), that were ALT-probability <0.75 (ALT-low) by Sieverling’s score; the blue shading in the lower box indicates tumors with ALT-low probability (new classifier), that were ALT-probability >0.75 (ALT-high) by Sieverling’s score. 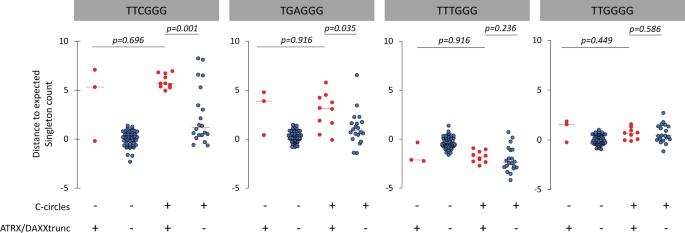Fig. 2: Distance to the expected singleton repeat count in tumors with negative C-circle assay, with (n= 3), or without (n= 58) ATRX/DAXXtrunc, and in tumors with positive C-circle assay with (n= 10), or without (n= 20) ATRX/DAXXtrunc. The center (horizontal) red line of the scattergrams is the median.p< 0.05 was considered as significant; Kolmogorov–Smirnov tests, two-tailed. Sieverling et al. [2] and Lee et al. [3] ALT-probability scores were compared using Spearman’s correlation. Distances to the expected singleton repeat count distributions [2] in tumors with negative CCA [3] , with or without ATRX/DAXXtrunc [2] , and in tumors with positive CCA [3] with, or without ATRX/DAXXtrunc [2] were compared using two-tailed Kolmogorov–Smirnov tests at the 5% level of significance. To develop a classifier, based on CCA data [3] as an indicator of ALT, we searched for the best combination signature associated with CCA status [3] within the genomic features and telomere content determined by Sieverling et al. with the Telomere Hunter WGS tool [2] (telomere content tumor/control log2 ratio, telomere insertion count, breakpoint count, and singleton distributions), using Akaike information criterion stepwise regression analysis. Statistical analyses were carried out using R version 3.6.2 (R Foundation for Statistical Computing). Reporting summary Further information on research design is available in the Nature Research Reporting Summary linked to this article.